Hard magnetic ferrite with a gigantic coercivity and high frequency millimetre wave rotation Magnetic ferrites such as Fe 3 O 4 and Fe 2 O 3 are extensively used in a range of applications because they are inexpensive and chemically stable. Here we show that rhodium-substituted ε-Fe 2 O 3 , ε-Rh x Fe 2− x O 3 nanomagnets prepared by a nanoscale chemical synthesis using mesoporous silica as a template, exhibit a huge coercive field ( H c ) of 27 kOe at room temperature. Furthermore, a crystallographically oriented sample recorded an H c value of 31 kOe, which is the largest value among metal-oxide-based magnets and is comparable to those of rare-earth magnets. In addition, ε-Rh x Fe 2− x O 3 shows high frequency millimetre wave absorption up to 209 GHz. ε-Rh 0.14 Fe 1.86 O 3 exhibits a rotation of the polarization plane of the propagated millimetre wave at 220 GHz, which is one of the promising carrier frequencies (the window of air) for millimetre wave wireless communications. Magnetic ferrite, which is composed of iron oxide, was discovered in the seventh century B.C. Since then, magnetic ferrites have contributed to daily life [1] , [2] , for example, magnetic motors, magnetic recording media, magnetic fluids and electromagnetic wave filters. However, due to their low magnetocrystalline anisotropies [3] , [4] , [5] , the coercivity of magnetic ferrites is generally low. Hence, the development of magnetic ferrites with a large coercive field ( H c ) is an important issue because this type of ferrite can be used as various advanced materials [6] , [7] , [8] . Of the several polymorphs of Fe 2 O 3 (refs 9 , 10 ), γ-Fe 2 O 3 and α-Fe 2 O 3 phases have been well studied. γ-Fe 2 O 3 , which is a representative soft magnet, is a ferrimagnet with a spinel structure. α-Fe 2 O 3 has a corundum structure and shows weak ferromagnetism due to the Dzyaloshinsky−Moriya mechanism [11] , [12] . In contrast, ε-Fe 2 O 3 is a rare phase, and research on this phase had been running behind [13] , [14] , [15] . It is only recently that ε-Fe 2 O 3 was found to exhibit a huge coercive field of 20 kOe at room temperature [16] . Since then, its magnetic properties have received much attention [17] , [18] , [19] , [20] , [21] . In this Article we synthesized rhodium-substituted ε-iron oxide, ε-Rh x Fe 2− x O 3 , nanomagnets and found that this series exhibits the highest H c value of 31 kOe among metal oxides. This H c value is comparable to those of rare-earth magnets [22] , [23] . Furthermore, it displays electromagnetic wave absorption with the highest resonance frequency among whole magnetic materials. Herein, we report the synthesis, crystal structure, magnetic properties, first-principles calculations, high frequency millimetre wave absorption properties and magnetic rotation of the propagated millimetre wave. Synthesis and crystal structure of ε-Rh x Fe 2− x O 3 nanomagnets A series of rhodium-substituted epsilon-iron oxide nanoparticles (ε-Rh x Fe 2− x O 3 , x =0, 0.04, 0.07, 0.11 and 0.14) were prepared by impregnating a methanol and water solution containing iron nitrate and rhodium nitrate into mesoporous silica, subsequently heating at 1,200 °C in air, and removing the silica matrix using an aqueous sodium hydroxide solution ( Fig. 1a ) (see Methods ). The transmission electron microscope image indicates that the obtained sample is composed of nanoparticles with an average particle size of ca. 35 nm (inset of Fig. 1a ; Supplementary Fig. S1 ). 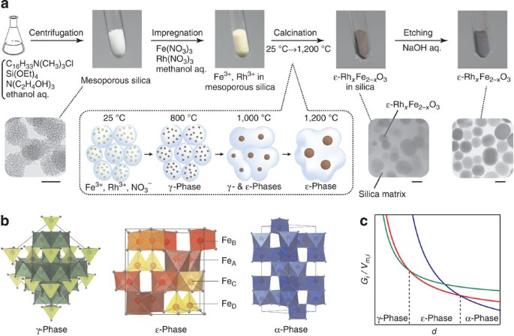Figure 1: Synthesis, crystal structure and thermodynamic stability of ε-RhxFe2−xO3nanomagnets. (a) Upper row illustrates the synthesis of ε-RhxFe2−xO3. In the first step, a mesoporous silica template is synthesized in a conical flask to give a white powder. In the second step, an aqueous solution of Fe(NO3)3and Rh(NO3)3with methanol is impregnated into the silica to yield a yellow powder. In the third step, the resulting product is calcinated in air, and in the fourth step, the final product is obtained after etching the silica matrix with an aqueous NaOH solution. Lower left transmission electron microscope (TEM) image shows the obtained mesoporous silica where the small white dots are the mesopores. Illustration in the dotted frame depicts the formation process of ε-phase during calcination; as the temperature increases, Fe(NO3)3and Rh(NO3)3in the mesopores turn into γ-phase (~800 °C). Around the melting temperature of glass (1,000 °C), the particles begin to aggregate. As shown in the centre TEM image, ε-phase is the main phase at 1,200 °C. Lower right TEM image is the final product after etching the silica matrix. The scale bars below the three TEM images indicate 30 nm. (b) (left) Crystal structure of γ-phase. Green and light green indicate octahedral and tetrahedral Fe sites, respectively. (centre) Crystal structure of ε-phase. Dark red, red, orange and yellow indicate the four nonequivalent Fe sites for FeA, FeB, FeCand FeD, respectively. (right) Crystal structure of α-phase. Fe site is shown as blue octahedrons. Grey lines indicate the unit cell. (c) CalculatedGi/Vm,iversusdcurves fori-phases (i=γ, ε and α). Green, red and blue curves correspond to γ-phase, ε-phase and α-phase, respectively. The curves are calculated under the condition ofμγ>με>μα,σγ<σε<σαand (σε−σγ)/(σα−σε) < (με−μγ)/(μα−με), whereμiis the chemical potential ofi-phase andσiis the surface energy ofi-phase. Figure 1: Synthesis, crystal structure and thermodynamic stability of ε-Rh x Fe 2− x O 3 nanomagnets. ( a ) Upper row illustrates the synthesis of ε-Rh x Fe 2− x O 3 . In the first step, a mesoporous silica template is synthesized in a conical flask to give a white powder. In the second step, an aqueous solution of Fe(NO 3 ) 3 and Rh(NO 3 ) 3 with methanol is impregnated into the silica to yield a yellow powder. In the third step, the resulting product is calcinated in air, and in the fourth step, the final product is obtained after etching the silica matrix with an aqueous NaOH solution. Lower left transmission electron microscope (TEM) image shows the obtained mesoporous silica where the small white dots are the mesopores. Illustration in the dotted frame depicts the formation process of ε-phase during calcination; as the temperature increases, Fe(NO 3 ) 3 and Rh(NO 3 ) 3 in the mesopores turn into γ-phase (~800 °C). Around the melting temperature of glass (1,000 °C), the particles begin to aggregate. As shown in the centre TEM image, ε-phase is the main phase at 1,200 °C. Lower right TEM image is the final product after etching the silica matrix. The scale bars below the three TEM images indicate 30 nm. ( b ) (left) Crystal structure of γ-phase. Green and light green indicate octahedral and tetrahedral Fe sites, respectively. (centre) Crystal structure of ε-phase. Dark red, red, orange and yellow indicate the four nonequivalent Fe sites for Fe A , Fe B , Fe C and Fe D , respectively. (right) Crystal structure of α-phase. Fe site is shown as blue octahedrons. Grey lines indicate the unit cell. ( c ) Calculated G i / V m ,i versus d curves for i -phases ( i =γ, ε and α). Green, red and blue curves correspond to γ-phase, ε-phase and α-phase, respectively. The curves are calculated under the condition of μ γ > μ ε > μ α , σ γ < σ ε < σ α and ( σ ε − σ γ )/( σ α − σ ε ) < ( μ ε − μ γ )/( μ α − μ ε ), where μ i is the chemical potential of i -phase and σ i is the surface energy of i -phase. Full size image The X-ray diffraction patterns confirm that the crystal structure is orthorhombic with Pna 2 1 space group ( Fig. 1b ). Rh substitutes for a specific iron site (Fe C site) among the four nonequivalent iron sites (Fe A –Fe D sites) in the crystal structure of ε-Rh x Fe 2− x O 3 . The unit cell volume refined by the Rietveld analysis gradually increases with Rh concentration. At higher Rh concentrations, α-Rh x Fe 2− x O 3 is formed as a byproduct ( Supplementary Fig. S2 and Supplementary Table S1 ). The particle size distribution depends on the sintering temperature; the particle size increases as the sintering temperature increases, and the phase changes from γ-phase to ε-phase and then to α-phase ( Fig. 1c ). The threshold sizes for the transformation from γ- to ε-phase and from ε- to α-phase are evaluated to be 10 and 55 nm, respectively ( Supplementary Fig. S3 ). Magnetic properties The magnetic properties were measured by a superconducting quantum interference device (SQUID) magnetometre. The temperature dependences of the magnetization of ε-Rh x Fe 2− x O 3 powder samples show that the Curie temperatures ( T C ) are 505 K ( x =0), 495 K ( x =0.04), 484 K ( x =0.07), 474 K ( x =0.11) and 469 K ( x =0.14) ( Supplementary Fig. S4a ). The magnetization versus external magnetic field plots at 300 K demonstrate that the H c value increases as the x value increases, that is, 22 kOe ( x =0), 23 kOe ( x =0.04), 24 kOe ( x =0.07), 25 kOe ( x =0.11) and 27 kOe ( x =0.14) ( Fig. 2a and Supplementary Fig. S4b ). 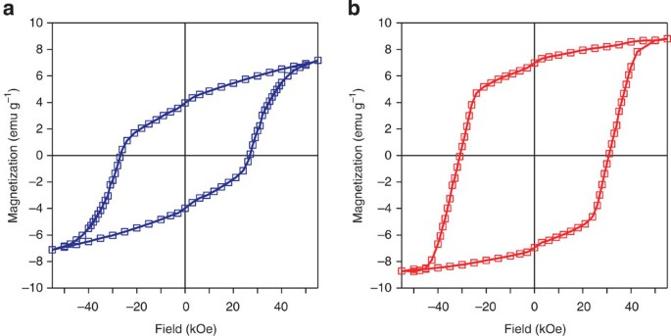Figure 2: Magnetic properties of ε-RhxFe2−xO3nanomagnets. (a) Magnetization versus external magnetic field plot of non-oriented ε-Rh0.14Fe1.86O3nanoparticles at 300 K exhibiting a coercive field of 27 kOe. (b) Magnetization versus external magnetic field plot of crystallographically oriented ε-Rh0.14Fe1.86O3/resin at 300 K exhibiting a coercive field of 31 kOe. Figure 2: Magnetic properties of ε-Rh x Fe 2− x O 3 nanomagnets. ( a ) Magnetization versus external magnetic field plot of non-oriented ε-Rh 0.14 Fe 1.86 O 3 nanoparticles at 300 K exhibiting a coercive field of 27 kOe. ( b ) Magnetization versus external magnetic field plot of crystallographically oriented ε-Rh 0.14 Fe 1.86 O 3 /resin at 300 K exhibiting a coercive field of 31 kOe. Full size image Furthermore, crystallographically oriented ε-Rh 0.14 Fe 1.86 O 3 nanoparticles dispersed in resin (see Methods ) reveal a gigantic H c value of 31 kOe ( Fig. 2b ), which is related to the magnetic anisotropy field ( H a ) as H c ≈ H a /2 with a uniaxial magnetic anisotropy. The magnetic hysteresis loop indicates that the estimated H a value of the sample for x =0.14 is 53 kOe, which is much larger than those of γ-Fe 2 O 3 (0.2 kOe) and Fe 3 O 4 (0.5 kOe). First-principles calculations First-principles calculations of ε-Rh x Fe 2− x O 3 were conducted to understand the electronic structure of this series (see Methods ). The density of states (DOS) shows that ε-Rh x Fe 2− x O 3 is a charge-transfer type insulator with an O2 p valence band and a Fe3 d conduction band ( Supplementary Fig. S5 ). Rh4 d is distributed in the same energy region as the O2 p band below the Fermi energy ( E F ) level, suggesting that Rh4 d and O2 p overlap greatly. In the occupied region, the 3 d bands of the Fe B and Fe C sites are occupied by α spins, whereas those of the Fe A and Fe D sites are occupied by β spins, that is, (Fe A , Fe B , Fe C , Fe D )=(β, α, α, β) ( Supplementary Fig. S6 ). Although we attempted several alternative spin configurations, their energies are higher than that of (β, α, α, β), suggesting that these other configurations are not suitable. This finding is consistent with the spin configuration reported for ε-Fe 2 O 3 , which is a collinear ferrimagnet composed of positive sublattice magnetizations at the Fe B and Fe C sites and negative sublattice magnetizations at the Fe A and Fe D sites [24] , [25] . The charge density map shows strong hybridization between Fe 3+ and O 2− ; the electron charge is partially transferred from O 2− to Fe 3+ through hybridization ( Supplementary Fig. S7 ). Millimetre wave absorption properties The electromagnetic wave absorption properties were measured under a zero-magnetic field at room temperature in the millimetre wave range (30–300 GHz) using terahertz time domain spectroscopy (THz-TDS) (see Methods and Supplementary Fig. S8 ). As shown in Fig. 3a , resonance frequencies ( f r ) are observed at 182 GHz ( x =0), 186 GHz ( x =0.04), 190 GHz ( x =0.07), 198 GHz ( x =0.11) and 209 GHz ( x =0.14). These f r values are the highest among all magnetic materials. The f r versus H c plot shows that the f r value proportionally increases with increasing H c (the inset of Fig. 3a ). Before this work, ε-Fe 2 O 3 exhibited the highest f r value of 182 GHz [26] . As for the quality of the absorption, the Q -factor of the absorption, which is expressed as Q = f r /Δ f , where Δ f is full width at half maximum, is evaluated to be 38 ( x =0), 20 ( x =0.04), 21 ( x =0.07), 19 ( x =0.11) and 17 ( x =0.14). 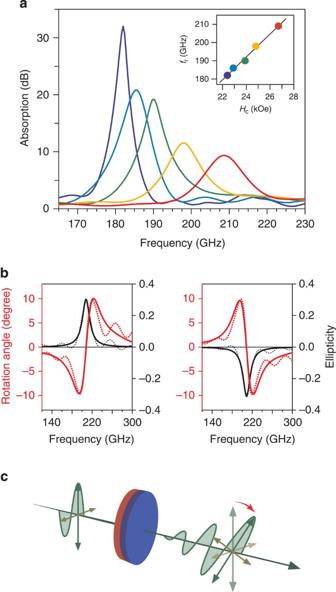Figure 3: Millimetre wave absorption and millimetre wave magnetic rotation of ε-RhxFe2−xO3nanomagnets. (a) Millimetre wave absorption spectra of ε-RhxFe2−xO3under a zero-magnetic field at room temperature forx=0 (blue),x=0.04 (light blue),x=0.07 (green),x=0.11 (orange) andx=0.14 (red) measured by THz-TDS. Inset plots the resonance frequency (fr) versus coercive field (Hc). Colours of the dots are consistent with thexvalues of the absorption spectra. Black line is to guide the eye. (b) Millimetre wave magnetic rotation and ellipticity change of ε-Rh0.14Fe1.86O3. Rotation angle (red dotted line) and ellipticity (black dotted line) spectra measured by irradiating from the N-pole side (left) and S-pole side (right) of the sample using THz-TDS. Solid lines are to guide the eye. (c) Schematic illustration of the magnetic rotation and ellipticity change of the propagated millimetre wave due to the optically induced magnetic dipole transition. The green and ochre arrows indicate the magnetic field and electric field components of the impulsive terahertz wave pulse, respectively. Red and blue sides of the disc denote the N- and S-poles of the magnetized pellet sample. Figure 3: Millimetre wave absorption and millimetre wave magnetic rotation of ε-Rh x Fe 2− x O 3 nanomagnets. ( a ) Millimetre wave absorption spectra of ε-Rh x Fe 2− x O 3 under a zero-magnetic field at room temperature for x =0 (blue), x =0.04 (light blue), x =0.07 (green), x =0.11 (orange) and x =0.14 (red) measured by THz-TDS. Inset plots the resonance frequency ( f r ) versus coercive field ( H c ). Colours of the dots are consistent with the x values of the absorption spectra. Black line is to guide the eye. ( b ) Millimetre wave magnetic rotation and ellipticity change of ε-Rh 0.14 Fe 1.86 O 3 . Rotation angle (red dotted line) and ellipticity (black dotted line) spectra measured by irradiating from the N-pole side (left) and S-pole side (right) of the sample using THz-TDS. Solid lines are to guide the eye. ( c ) Schematic illustration of the magnetic rotation and ellipticity change of the propagated millimetre wave due to the optically induced magnetic dipole transition. The green and ochre arrows indicate the magnetic field and electric field components of the impulsive terahertz wave pulse, respectively. Red and blue sides of the disc denote the N- and S-poles of the magnetized pellet sample. Full size image Magnetic rotation of the propagated millimetre wave The rotation angle and ellipticity were measured under a zero-magnetic field using a magnetized ε-Rh 0.14 Fe 1. 86 O 3 pellet sample, which was obtained by a strong pulsed magnetic field ( ca. 8T). Irradiating with a millimetre wave from the N-pole side of the sample causes the rotation angle to display a dispersive spectrum centred at f r =209 GHz where the minimum and maximum values are −10° and +10° at 196 and 220 GHz, respectively, whereas the ellipticity exhibits a peak at f r with a value of +0.3 ( Fig. 3b , left). Upsetting the magnetic poles of the sample inverts the signs of the rotation angle and ellipticity ( Fig. 3b , right). The observed phenomenon clearly originates from the remanent magnetization and its direction ( Fig. 3c ). The figure of merit ( F ), which is defined as F =(rotation angle (deg))/(absorption (dB)), has a high value of 20 deg dB −1 at 220 GHz. Usually, iron oxide (Fe 2 O 3 ) transforms directly from γ-phase into α-phase as the sintering temperature increases in the typical calcination process. However, in the present synthetic method, ε-phase exists as a stable phase due to the nanosize effects on the phase transformation via the following mechanism. In a nanoparticle, the free energy of each i -phase ( G i , i =γ, ε, or α) is expressed as the sum of the chemical potential ( μ i ) and surface energy ( A i σ i ), where A i and σ i represent the molar surface area and the surface free energy of the particle, respectively [27] ; G i = μ i + A i σ i . Because A i is equal to 6 V m, i / d , where V m, i and d represent the molar volume and particle diameter, respectively, the free energy per molar volume ( G i / V m, i ) is expressed as G i / V m, i = μ i / V m, i +6 σ i / d . This equation suggests that the surface energy contribution increases as the particle diameter decreases. When the parameters in the equation satisfy the relationships of μ γ > μ ε > μ α , σ γ < σ ε < σ α and ( σ ε − σ γ )/( σ α − σ ε ) <( μ ε − μ γ )/( μ α − μ ε ), then the curves for G γ / V m,γ , G ε / V m,ε and G α / V m,α intersect, leading to the stable ε-phase at an intermediate d value ( Fig. 1c ). Such a nanosize effect has also been reported in Al 2 O 3 (refs 28 , 29 ) and Ti 3 O 5 (ref. 30 ). Next, we considered the mechanism of the large H c value in the present material. One origin of the gigantic H c is that the particle size of ca . 35 nm in the present series should be sufficiently small to form a single magnetic domain [3] , [31] . In fact, the magnetic force microscopy image for x =0 shows that each particle has a single magnetic domain (see Methods ). In a single magnetic domain, only the magnetization rotation process operates, leading to a large H c value. Another origin of the gigantic H c is the magnetic anisotropy of the ε-phase. Because shape anisotropy in the present series is negligible (below 0.3 kOe), the observed H a value of 53 kOe is determined by the magnetocrystalline anisotropy. The results of the first-principles calculations indicate that the following mechanism explains the large magnetocrystalline anisotropy of this series. The charge density map ( Supplementary Fig. S7 ) shows strong hybridization between Fe 3+ and O 2− , that is, the electron charge is partially transferred from O 2− to Fe 3+ , resulting in an electron configuration of d 5+ q where q is the transferred charge. Such a hybridization causes a non-zero orbital angular momentum ( L ≠ 0) on Fe ion, which induces a large magnetocrystalline anisotropy. Furthermore, Rh–O–Fe hybridization is observed around the Rh-substituted site, which enhances the magnetocrystalline anisotropy through the contribution from the orbital angular momentum on Rh. Thus, the large H c value of the present material is attributed to the nanoscale particle size, which is suitable to form a single magnetic domain, and the huge H a value due to the magnetocrystalline anisotropy. Finally, we discuss millimetre wave absorption, magnetic rotation and ellipticity change of the propagated millimetre wave. In a ferromagnetic material with a uniaxial magnetic anisotropy, an electromagnetic wave is absorbed at f r , known as zero-field ferromagnetic resonance (natural resonance). Because the magnitude of the H a value determines the f r value, that is, f r = νH a /2π, where ν is the gyromagnetic constant, the observed high f r values are due to the large H a values of ε-Rh x Fe 2– x O 3 . In fact, the f r versus H c plot shows that the f r value proportionally increases with increasing H c ( Fig. 3a ). Furthermore, zero-field ferromagnetic resonance generates changes in the rotation angle and ellipticity of the propagated millimetre wave. When an impulsive terahertz wave pulse is irradiated into the sample, the magnetic field component of the terahertz wave tilts the spontaneous magnetization away from the magnetic easy-axis direction due to gyromagnetic effect, which causes the bulk magnetization to precess around the easy axis. This precession produces a magnetic rotation of the propagated millimetre wave at a particular frequency ( Fig. 3c ; Supplementary Movie 1 ). These observed millimetre wave absorption, magnetic rotation and ellipticity change are due to the optically induced magnetic dipole transition, which differs from the conventional magneto–optic effect (Faraday effect) in the visible or near-infrared region through an optically induced electric dipole transition [32] . In conclusion, we prepared a series of ε-Rh x Fe 2− x O 3 nanomagnets via a nanoscale synthetic method using mesoporous silica as a template. ε-Rh 0.14 Fe 1.86 O 3 displays the largest H c value of 31 kOe among metal-oxide magnets. The gigantic H c value has potential in future high-density magnetic recording media because the large H c value enables the particle size to be greatly reduced while maintaining coercivity. In addition, ε-Rh x Fe 2− x O 3 exhibits a zero-field ferromagnetic resonance up to 209 GHz, and the magnetic rotation and ellipticity change of the propagated millimetre wave occur due to an optically induced magnetic dipole transition at 220 GHz. The present material should be useful for high frequency millimetre wave absorbers and rotators (isolators or circulators) as it should restrict electromagnetic interference problems [33] because the frequency of the magnetic rotation corresponds to the highest window of air (220 GHz band), which is the anticipated carrier frequency for next-generation millimetre wave wireless communications such as high-definition television communications and intra-board integrated circuit (IC) chip wireless communications [34] , [35] , [36] . Materials An impregnation method using mesoporous silica nanoparticles was used to prepare a series of ε-Rh x Fe 2− x O 3 ( x =0, 0.04, 0.07, 0.11 and 0.14) nanoparticles. Mesoporous silica nanoparticles were synthesized by modifying reported methods [37] , [38] . Tetraethyl orthosilicate (62 mmol) was added to a solution of distilled water (4 mol), ethanol (0.18 mol), cetyltrimethylammonium chloride (16 mmol) and triethanolamine (62 mmol) at 60 °C, yielding mesoporous silica nanoparticles after centrifuging and heating at 600 °C in air. To obtain the target materials, a methanol and water solution containing iron nitrate and rhodium nitrate was immersed into mesoporous silica and sintered at 1,200 °C for 4 h in air. Silica matrices were etched by an aqueous sodium hydroxide solution at 70 °C. Physical property measurements Elemental analyses of the prepared samples were conducted with inductively coupled plasma mass spectroscopy (Agilent Technologies, HP 4500). Transmission electron microscope images were acquired with JEM 2000EX. The 2 θ – θ scan X-ray diffraction measurements were performed using Rigaku Ultima IV and Rigaku RINT2100 with Cu Kα radiation ( λ =1.5418 Å) at 293 K. Rietveld analyses were performed using the RIETAN-FP program [39] . The magnetic properties were measured using a SQUID magnetometer (Quantum Design, MPMS 7). Preparation of an oriented sample An oriented ε-Rh 0.14 Fe 1. 86 O 3 /resin was prepared. The ε-Rh 0.14 Fe 1.86 O 3 nanoparticles were oriented by placing ε-Rh 0.14 Fe 1.86 O 3 nanoparticles dispersed ultraviolet curing resin (SD-2200, DIC Corporation) in an applied magnetic field of 12.7 kOe. The sample was then irradiated with ultraviolet light (EX250, Hoya Candeo Optronics Corporation) to harden the curing resin and to pin the oriented nanoparticles. Single magnetic domain of the nanoparticle With respect to the magnetic domain, we previously performed magnetic force microscopy measurements on ε-Fe 2 O 3 , which was prepared by a combination of reverse-micelle and sol–gel methods. The magnetic force microscopy image showed that ε-Fe 2 O 3 particles form a single magnetic domain. Therefore, ε-Rh x Fe 2− x O 3 is considered to be composed of a single magnetic domain. Additionally, the magnetic domain sizes of common metal-oxide–based magnets are much larger than the size of our nanoparticles. For example, the magnetic domain size of barium ferrite is about 1 μm [40] . First-principles calculations First-principles calculations were performed using Vienna ab initio Simulation Package, which is a plane–wave projector augmented wave method program [41] , [42] . The exchange-correlation functional was approximated with generalized gradient approximation (GGA) parameterized by Perdew–Burke–Ernzerhof (PBE) in the spin-restricted condition. To describe the Fe3 d and Rh4 d orbitals, the Hubbard U term (GGA+ U ) was considered. Referring to the reported calculations for α-Fe 2 O 3 and γ-Fe 2 O 3 , the difference between the Coulomb interaction energy ( U coul ) and exchange interaction energy ( J ex ), U coul − J ex , was set to 4.0 eV. The basis set size was regulated by a cutoff energy of 520 eV. Gaussian methods (smearing width: 0.2 eV) were used to integrate the Brillouin zone with a 3×3×3 k -mesh and to calculate the DOS with a 5×3×3 k -mesh. Among the 16 Fe atoms in the unit cell, a Rh atom substituted for one Fe atom at the Fe C site. Supplementary Figures S5–S7 show the calculated DOS and charge density map. Millimetre wave absorption measurements A pump-probe measurement system was used for the THz-TDS measurements. Supplementary Figure S8 schematically diagrams the THz-TDS system. A mode-locked Ti:sapphire pulse laser delivered 20-fs long ultrashort light pulses with a central photon energy of 1.55 eV at a pulse repetition rate of 76 MHz. A beam splitter divided the output of the mode-locked Ti:sapphire femtosecond pulse laser into pump and probe beams. Dipole type and bowtie type low-temperature-grown GaAs photoconductive antennas were used as the THz wave emitter and detector, respectively. The emitted THz wave was collimated and irradiated into the sample, which was mounted on a sample holder and placed between a set of paraboloidal mirrors. The transmitted THz electric field was detected with the bowtie type low-temperature-grown GaAs photoconductive antenna, which was triggered by optical probe pulses with variable time delays between the pump and probe pulses; consequently, the electric field of the transmitted THz pulse wave was formed in the time domain. The absorption spectra of the THz waves were calculated as (Absorption)=−10 log | t ( ω )| 2 [dB], where t ( ω ) is the complex amplitude transmittance. Samples were held in paper containers with filling factors of ca. 30%. Millimetre wave magnetic rotation measurements To obtain the millimetre wave magnetic rotation spectra, we employed three polarizers (P1–P3) to measure the horizontal and vertical polarization components ( Supplementary Fig. S8 ). The measurement system operated only the horizontal polarization component of the electric field because the antenna determined the directions of the THz wave emitter and detector. To precisely define the polarization of the THz wave as horizontal (0°), P1 was placed after the emitter while P3 was placed before the detector. The components of +45° and −45° were measured by rotating P2 behind the sample. The vertical and horizontal polarization components were obtained as their difference and sum, respectively. The rotation angle and ellipticity were obtained from the horizontal and vertical components ( E x ( t ), E y ( t )) of the transmitted electric fields, which are expressed as The rotation angle φ ( ω ) and ellipticity η ( ω ) spectra are expressed as where δ ( ω )= δ 1 ( ω )− δ 2 ( ω ) is the phase difference. a ( ω ) and η ( ω ) can be directly determined as the Fourier-transformed amplitude and phase of the temporal waveforms. How to cite this article: Namai, A., et al . Hard magnetic ferrite with a gigantic coercivity and high frequency millimeter wave rotation. Nat. Commun. 3:1035 doi: 10.1038/ncomms2038 (2012).